(NHC)Pd(II) hydride-catalyzed dehydroaromatization by olefin chain-walking isomerization and transfer-dehydrogenation Transition-metal-catalyzed homogeneous dehydrogenation and isomerization are common organic molecular activation reactions. Palladium hydrides are good olefin isomerization catalysts but are usually short-lived species under redox-active dehydrogenation conditions. Here, we show that Pd-H in the presence of an N-heterocyclic carbene ligand and an alkene regulator enables transfer-dehydroaromatization, avoiding the homo-disproportionation pathway. The desired product is obtained with up to 99:1 selectivity, and the exo-to-endo olefin isomerization can be carried out in one pot. In contrast to previously reported methods that rely on the efficient removal of Pd-H, the approach reported herein benefits from the steric effects of the N-heterocyclic carbene and the choice of alkene to regulate the competing reactivity of allylic C‒H activation and hydropalladation. This method circumvents the challenges associated with tedious olefin separation and a low exo-to-endo olefin isomerization ratio and expands the scope to include challenging endo- and exo-cyclic olefins under mild, neutral, and oxidant-free conditions. Overall, herein, we provide a strategy to synthesize (hetero)aromatic compounds via chemoselective dehydrogenation of cyclic alkenes over ketones and the dehydrogenative Diels-Alder reaction of a cyclic enamine. Dehydrogenation (DH) [1] , [2] , [3] , [4] and chain-walking functionalization [5] , [6] are two essential strategies for molecular activation. These methods add value to abundant natural resources, such as carbonyls, alkenes, Diels-Alder adducts, and alkanes [7] . In particular, DH of cyclic compounds by transition-metal catalysis has long been vital for aromatic compound synthesis [8] , [9] , [10] , [11] (Fig. 1a , dehydroaromatization (DHA)) [12] , [13] , [14] , [15] , [16] , [17] , [18] . Transition-metal hydrides are common intermediates in catalytic cycles. A longstanding fundamental challenge has been the precise control of transition-metal hydride behavior; otherwise, disproportionation and hydrometallation often limit the yield and efficiency of this process. Certain innovative approaches, such as the use of Ir, Pt, Cu, and Pd catalysts with pincer and diimine ligands [7] , [19] , [20] , [21] , [22] , [23] , [24] , as well as Pd/C heterogeneous systems, have been developed to eliminate unproductive hydrometallation that can cause undesired transformations or slow catalyst regeneration. Some of these schemes can be implemented by using inexpensive oxidants or O 2 for the efficient removal of M-hydrides (Fig. 1b, c ) [20] , [25] , [26] , [27] . Photoredox-active transition-metal catalysis can be used to effectively prepare naphthalenes and N-heterocycles at r.t. [28] , [29] , where less activated cyclohexenes have not yet been utilized as good substrates (Fig. 1d ). An alkene can be used as a gaseous H 2 acceptor to enable DHA of 1,3-diones and cyclohexa-1,4-dienes catalyzed by Pd/C [30] , [31] , B(C 6 F 5 ) 3 [32] and alkaline-earth metals [33] at 60–130 °C. However, the aforementioned powerful strategies also completely block some desired functions of transition-metal hydrides, such as olefin isomerization. Some conditions, such as high temperature and highly redox-active environments, limit the substrate scope to specific endocyclic olefins. Many exocyclic olefins that can be accessed easily from either natural resources or standard 1,n-diyne/diene cycloisomerizations have not yet been utilized as ideal substrates. It is challenging to develop a dual-function catalyst or to combine two catalysts in one pot to carry out both exo-to-endo alkene isomerization and DH. Different redox potentials of the catalysts and reagents may negatively affect the desired elementary steps. Branched and conjugated exocyclic olefins may result in additional complications, such as a high styrene-to-ethylbenzene ratio that is frequently observed when using 4-vinyl-cyclohexene, as well as subsequent hydrogenation by high-pressure steam to afford high ethylbenzene selectivity [34] . The high relative yield of the styrene product also implies that the Pd-H generated in the redox-active catalytic cycle is short-lived. Fig. 1: Strategies in Pd-Catalyzed Dehydroaromatization (DHA). a Conventional dehydroaromatization. b Pd-H recycled/removed by O 2 . c AMS/quinone-assisted Pd(II) regeneration. d Photoredox catalytic cycles via thiyl radicals. e NHC-Pd-H directed transfer-dehydroaromatization. Full size image In this work, instead of developing more practical Pd-H removal methods by oxidation or reductive elimination, we employ an alternate strategy that relies on the conservation of Pd-H. Herein, NHC [35] stabilizes Pd(II)H to perform transfer-dehydroaromatization (TDHA) for several challenging exo- and endocyclic olefins under mild and neutral conditions (Fig. 1e . endo- at r.t.; exo- at 50–70 °C, without a strong oxidant or cocatalyst). Unlike approaches based on fast Pd(II)H removal by an oxidant/acid/base, the desired olefin isomerization and DH can be carried out simultaneously in one pot facilitated by suitable selections of NHC L and regulator R (Fig. 2 ). This dynamic combination provides an efficient way to control hydropalladation vs. allyl DH for a broad range of exo- and endo-olefins. Fig. 2: N-Heterocyclic carbene L and regulator R employed in this study. a NHC L1-7 structures . b Regulator R1-9 structures. Full size image Catalyst development and optimization An unexpected discovery resulted from our continuing efforts to use an NHC-ligated transition-metal hydride to catalyze olefin cross-hydroalkenylation [36] , [37] , [38] . An in situ-generated Pd(II)H catalyst was prepared from PdCl 2 /NHC/HSi(OEt) 3 , characterized by 1 H NMR, and used instead of an (NHC)Ni(allyl)X catalyst to afford a notable quantity of product 2a from endocyclic olefin 1a and α-olefin R1 [10] (Fig. 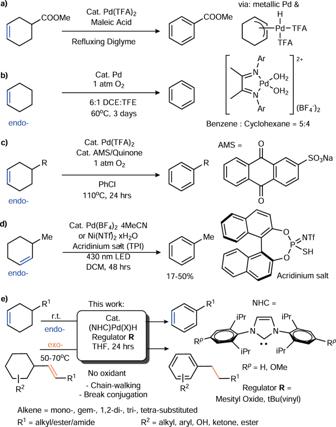Fig. 1: Strategies in Pd-Catalyzed Dehydroaromatization (DHA). aConventional dehydroaromatization.bPd-H recycled/removed by O2.cAMS/quinone-assisted Pd(II) regeneration.dPhotoredox catalytic cycles via thiyl radicals.eNHC-Pd-H directed transfer-dehydroaromatization. 1e , Table 1 , Entry 1), and no cross-hydroalkenylation of 1a and R1 was observed even when the catalyst was treated with NaBArF ( 1a conv. 45%, 24% 2a , 19% 4a ). The reaction was carried out simply under N 2 in THF at r.t. in the presence of a catalytic quantity of a reductant rather than the stoichiometric quantity of an oxidant used for related CH activations (i.e., HSi(OEt) 3 vs. PhIX 2 , Br 2 , CuCl 2 , or O 2 ), in sharp contrast to the elegant redox-active catalytic cycles based on the reoxidation of Pd species by a common oxidant [Pd(0→II) [20] , [21] ; Pd(II→IV) [39] , [40] ] [41] , [42] , [43] , [44] , [45] . Indeed, control experiments (Entries 2 and 3) further showed that our reaction did not proceed effectively in O 2 or without HSi(OEt) 3 . No oxidation of olefin 1a to the corresponding alcohol/ketone was detected. Thus, the catalytic formation of 2a did not involve the sequential dehydration of a Wacker-oxidation product in the presence of NHC/PdCl 2 /THF/O 2 [46] , [47] , and allylic alcohols were not intermediates in the mechanism. This conclusion was supported by the successful formation of the phenol product and the lack of formation of the arene product (benzene) from allylic alcohol (2-cyclohexenol) and 3-cyclohexenol ( 1e ) under standard conditions (as detailed below). The formation of an (NHC)Pd(II)H intermediate species was also supported by the detection of disproportionation product 3a and olefin isomerization product 4a . These observations revealed a unique opportunity to convert a mechanism consisting of undesired disproportionation [9] (e.g., 4- t -butyl-cyclohexene disproportionation mediated by Pd(TFA) 2 in the absence of an external oxidant, which was attributed to the loss of H-TFA) and hydropalladation into the desired TDHA mechanism with optimal isomerization under mild and neutral conditions. Here, we hypothesize that the steric effect of NHC may enable the desired chemoselective transfer-DH and isomerization reactivity (Fig. 3 ). Furthermore, the electronic effect of NHC may suppress the undesired Pd(X)H reductive elimination to a metallic Pd(0) species. In particular, the reversible and chemoselective hydropalladation ability of the relatively more stable (NHC)Pd(II)H may catalyze olefin isomerization, as well as allyl DH, by forming an alkyl-Pd(II) species similar to Me-Pd(II)/Pt(II) [22] . Table 1 Optimization of (NHC)Pd(II) catalyzed transfer-dehydroaromatization (TDHA) Full size table Fig. 3: Catalytic action of (NHC)Pd(II)H. a Cooperative steric effects of NHC and the alkene enable interchangeability of the Pd(II)H reactivity. b Conversion of a mechanism consisting of undesired disproportionation and hydropalladation into the desired TDHA mechanism. Full size image The analysis presented above shows that the selection of substituents on R is crucial for achieving a good yield and a high 2 : 3 ratio (Fig. 2 ). Screening for acyclic alkene R confirmed that R1 is not a molecular H 2 acceptor [10] , [30] . Replacing R1 with other simple α-olefins, such as 1-octene or aromatic olefins, resulted in a low conversion of 1a and afforded the 1-octene isomerization product (Entries 4–6). These findings suggested that the isomerization reactivity of a linear olefin is highly competitive and that the hydropalladation of aromatic alkenes may limit the desired reactivity by benzylic stabilization (see below for the solution to this problem and its application). Using cyclic olefins with allyl CH as R (such as 1a itself and cyclohexene ( R5 )) resulted in a shift in the product selectivity. 3a was favored over 2a , and ~50% benzene based on R5 was produced (see Entries 7 and 8, c.f. 1, respectively). This set of results suggested that the undesired reduction of 1a could be favored if an unsuitable R group was selected and that the ester moiety in 1a is not an essential directing group for the desired reactivity. Norbornene R6 , an excellent hydropalladation substrate that only contains a bridgehead allyl CH, was expected to be an excellent R group that would prevent 1a homodisproportionation. However, R6 exhibited only very limited reactivity (Entry 7 vs. Entry 9), possibly due to strong steric repulsion. In addition to R1 , acyclic carbonyl-activated olefins are also possible, albeit less efficient, choices for R for this reaction (Entries 10-12). Overall, the structural features and properties of R were identified as the controlling factors for the desired reactivity and selectivity. Screening of NHC revealed its critical role in this reaction as well (Fig. 2 , Table 1 , Entries 13-18). The choice of ligand was expected to be very important because cyclohexene is a common sacrificial olefin that produces Pd(II)H from (dcpe)Pd(II)Me for isomerization [48] . In the presence of NHC (Entries 1 and 13–18), the desired reactivity and high selectivity were generally observed. In contrast, the desired reactivity was not observed in the absence of NHC, even when R1 and silane were used (Entry 19). The most significant advance was realized by adding an electronic activator at the N-aryl p-position of NHC (Entry 1 vs. Entry 15), where an electron donor was found to be the most effective ( L4 ). Placing additional steric pressure at the core ( L2 ), N-aryl p-position ( L5 ), and o-position ( L7 ) of NHC caused the reactivity to decrease. The enhanced performance obtained by using L4 was attributed mainly to the increased σ-donating ability of NHC [49] , [50] and partly to the optimal steric effect either at the NHC V% bur [51] , [52] or the N-aryl p-position, since the donor may stabilize Pd(II)H against undesirable reductive elimination to Pd(0) and increase the hydropalladation selectivity (where the olefin R1 is less electron-rich and smaller than 1a ). Adding R1 to the reaction remains important even when using the electronically and sterically optimized NHC L4 ; otherwise, homodisproportionation remains the main pathway for DH (Entry 20). This result confirmed that the concomitant use of a hydride and R1 with NHC/PdCl 2 is key to achieving the desired reactivity and suggested that the direct DH of 1a by (NHC)Pd(II)H to produce H 2 is quite slow at r.t. Based on our hypothesis, the desired reactivity should be obtainable from other precatalyst combinations that can produce (NHC)Pd(II)H; thus, we also explored the use of L1 /Pd(TFA) 2 /HBpin (Entry 21). The reaction was catalyzed under the same physical conditions, as expected. This result did not correspond to background DH caused by Pd(TFA) 2 because a considerably lower reactivity was observed in the absence of HBpin (Entry 22). Comparing the results obtained using the two systems showed that the silyl and Bpin groups are not actively involved in the catalytic cycle. These combinations may be useful for expanding the substrate scope or precatalyst combinations based on differences in the steric and electronic properties of the respective compounds. However, L4 is not a good choice for Pd(TFA) 2 /HBpin. A significant decrease in the DH-to-isomerization ratio was observed (Entry 15 vs. Entry 23). Scope of endocyclic and exocyclic olefin TDHA With this basic information in hand, other endocyclic olefins were tested (Fig. 4 ). Several substrates with other functional groups and substituents were generally tolerated under the standard neutral condition with L4 at r.t. (Fig. 4a ) [21] , such as those substrates that can be obtained easily from Diels-Alder reactions (e.g., alkenyl ester/amide/Bpin/ether and dienes that afford 1a / 1b / 1c / 1f ). No apparent decrease in the catalytic reactivity was observed even with a cyclohexene containing an acid-sensitive epoxide ( 1f ). Phenol can be produced directly from a cyclohexenol ( 1e ), an epoxide ( 1f ) and an α,β-unsaturated ketone ( 1g ) [15] , [53] without the use of a protective or trapping group for OH. Moreover, aza-/oxa-heteroaromatics can be produced from endocyclic allyl-/vinyl-N/O (Figs. 4b , 1h-k ). The 2 : 3 ratio was increased by using an allyl carbamate instead of an amine ( 1j and 1 k ). Although elegant procedures have been developed for fused piperidine DH [28] , [54] , [55] , [56] , [57] , [58] , an N-substituted pyrrole ( 2i ) was easily obtained instead of an N-oxide under our oxidant-free conditions. As conjugated dienes are formed as conspicuous intermediates before the final DHA step, the typical condition with R1 remains effective (Fig. 4c ). Fig. 4: Endocyclic olefin 1 transfer-dehydroaromatization. a Cyclohexenes. b Heterosubstituted rings. c Dienes. d Fused rings. e Trisubstituted alkenes. Standard conditions: The olefin (0.25 mmol), L4 /PdCl 2 catalyst (0.025 mmol), HSi(OEt) 3 (0.0375 mmol), and R1 (0.5 mmol) were stirred in 2 mL of THF for 24 hrs at r.t. except if otherwise indicated. The yields of 2 and 2 : 3 (shown in parentheses) were determined by 1 H NMR (average of two runs). a 48 h; b as determined by GCMS (see the Supplementary Information for details); c the standard condition shown in Fig. 5 was used; d poor material balance due to a low b.p. ; e conversion, 1o : 83; 47; 100%; 1p-q : 25; 75; 89%; f 50 °C. Full size image The key advantage of our protocol is the use of logical combinations of NHC, X (e.g., TFA/Cl) and R to adapt to the structural characteristics of the substrate. Thus, a wide range of challenging alkenes can be used rather easily by simple modifications of the standard protocol. For instance, the relative hydropalladation efficiency between R and the substrates can be fine-tuned by a suitable choice and quantity of R . This selection can be guided by the literature on standard cross-hydroalkenylation (e.g., styrene is a better olefin acceptor than α-olefin in Ni(II)H-catalyzed cross-hydroalkenylation due to benzylic stabilization) [36] , [51] , [59] , thereby alleviating problems such as the low conversion and 2 : 3 ratio caused by the stabilization of the Pd(II) center after undesired hydropalladations at benzylic or tertiary carbon positions. Replacing R1 in the aforementioned standard protocol with aromatic olefin R4 and electronically activated trisubstituted olefin R8 (mesityl oxide, which is an inexpensive, low-boiling-point, and activated trisubstituted olefin that is removable by vacuum) restored the high 2 : 3 ratio and reactivity at 50 °C by reacting a fused aromatic olefin and a trisubstituted olefin with L1 (Fig. 4d, e , 1o , 1p , and 1q ). Replacing R1 with R8 in the initial condition including L1 resulted in a larger reduction of 1a ( 2a : 3a = 71:29 vs. 96:4 in Table 1 , Entry 11 vs. Entry 1), showing that R8 is a less effective hydropalladation substrate than the disubstituted alkene 1a ; thus, it is unlikely that the successful result shown in Fig. 4e involved a tri-to-disubstituted olefin isomerization ( 2 : 3 = 90:10) mechanism. One of the most remarkable aspects of this discovery is the ability of the NHC-Pd hydride to facilitate both olefin isomerization and TDHA in one pot for a suitably chosen R . The DH of 4-vinylcyclohexene has often been reported to produce a mixture of styrene and ethylbenzene in low yield and with low selectivity (41% and 14%, respectively) [24] . Our dual-function catalytic system limits undesired disproportionation, enables chain-walking alkene isomerization, and expands the substrate scope to many exocyclic olefins with diverse structural characteristics (Fig. 5 ). In general, reasonably high yield and selectivity were achieved using L1 /Pd(TFA) 2 /HBpin/ R8 at 50 °C instead of L1 /PdCl 2 /HSi(OEt) 3 , probably by altering the isomerization reactivity. Exocyclic olefins with diverse structural characteristics, e.g., methylene-, vinyl- and allyl-olefins with different degrees of substitution, including tri-/tetra-substituted olefins generated by chain walking, are all compatible (Fig. 5a ). R4 was used (Fig. 5b ) rather than R1 and R8 to address a similar challenge related to aromatic substituents, as previously discussed ( 1o in Fig. 4d ), to produce fused (hetero)arenes in both a high yield and 2′ : 3′ ratio, as predicted. Remarkably, as suggested by the R8 structural features, this method is also applicable to certain exocyclic α , β -conjugated carbonyl systems by disrupting the conjugation (Fig. 5c ). This ability is expected to be useful in combination with [(allyl)Pd(II)Cl] 2 -catalyzed α,β-DH of an ester/amide [60] , [61] system to develop a one-pot synthesis of an aromatic product under appropriate conditions. Moreover, the good functional group tolerance of the system is maintained. Substituents such as OH, COOMe, and CONHEt were found to be compatible, and no trans-esterification was observed ( 1′s, 1′r , and 1′n in Fig. 5c ). However, the 2′ : 3′ ratio decreased when tBu was replaced with a Ph group, showing that the decrease in the 2 : 3 ratio in the Ph case was likely caused by styrenyl formation ( 1′p and 1′q in Fig. 5c vs. 1o in Fig. 4d ) and not steric hindrance. R8 is an optimal R group for both trisubstituted endocyclic olefins and exocyclic systems. This result suggests that trisubstituted olefin is a common starting point for the desired TDHA. However, the generally higher yield and 2′ : 3′ ratio obtained from conjugated systems indicate that the carbonyl group may offer a more acidic allyl CH for direct activation. In addition to substituted methylene-cycloalkane structures accessible via typical 1,6-diene cycloisomerization, unsymmetrical 1,7-diene/diyne cycloisomerization products are also effective substrates for this system at 70 °C (Fig. 5d ). Fig. 5: Exocyclic olefin 1′ transfer-dehydroaromatization. a Aliphatic exocyclic olefins. b Fused aromatic rings. c Exo-conjugated systems. d Unsymmetric cycloisomerization products. Standard conditions: The olefin (0.25 mmol), L1 /Pd(TFA) 2 catalyst (0.025 mmol), HBpin (0.0375 mmol), and R8 (0.5 mmol) were stirred in 2 mL of THF for 24 h at 50 °C, unless otherwise indicated. The yields of 2 and 2 : 3 (shown in parentheses) were determined by 1 H NMR (as the average of two runs). a 48 h; b as determined by GCMS (see the Supplementary Information for details); c 60 °C; d 2.5 equiv. of R1 ; e Other products are from olefin isomerization; f 3 equiv. of R8 ; g 70 °C; h with a 9% aromatic product without OH. Full size image Replacing R8 with β -monosubstituted ketones ( R7 / R9 ) in our modular system enables the catalytic synthesis of substituted aniline and Diels-Alder derivatives from the corresponding enamine 1″a (Fig. 6 , c.f. 2″a:3″a ~37:63 with R8 ; ~50:50 with R1 , 10 mol% of base, where no DH background was observed in the absence of our catalyst). These successful results were notable for easily bypassing highly competitive reactions (e.g., Michael addition and cyclic amine DH) and enabled identification of the preferred allyl DH site for our catalyst. Note that although R7 (BQ) is a stoichiometric oxidant that is frequently used in several redox-active DH systems, the dehydrogenative Diels-Alder product has rarely been observed when using R7 . Hence, under redox-neutral and mild conditions with NHC, it is now possible to trap the in situ-generated endocyclic diene using challenging dienophiles or carry out other useful reactions, and the molecular complexity can be appropriately increased, as for acyclic diene systems [62] . This reaction sequence complements other one-pot reactions that primarily rely on aromatization first [63] . Fig. 6: Catalytic synthesis of a substituted aniline and dehydrogenative Diels-Alder product. a Synthesis of a substituted aniline. b Trapping the diene for the Diels-Alder reaction. Full size image A lower operating temperature, a broader substrate scope, and a higher isomerization ability than those of several well-known systems based on simple Pd(TFA) 2 were demonstrated for the proposed NHC system (e.g., 1a at r.t., c.f. 162 °C in maleic acid [9] and 105 °C in AMS/PhCl [21] ). While the current system was compatible with several known inhibitors [9] and useful for exocyclic olefins 1′ at ~50 °C, reported Pd(TFA) 2 systems afforded a <5% yield upon applying the known conditions to exocyclic olefins 1′o and allylcyclohexane, with or without NHC. These results prompted us to investigate the functions of NHC, silane/borane, and alkene R . First, the functions of silane/borane were studied. It might be reasonable to attribute the isomerization to the trace quantity of acid in the system (c.f. limonene isomerization by HCl/TFA [64] ), which was obtained via X-Si(OEt) 3 /-Bpin hydrolysis during catalyst generation or the reductive elimination of H-PdX [9] . However, adding a bulky organic base (2 equiv.) [64] to our system did not affect the desired reactivity (Fig. 7a ). Fig. 7: Control experiments and mechanistic studies. a Exocyclic olefin DHA using excess base. b Using [( L1 )PdCl( R )] 2 as an initiator in a mimic of the CH activation step at 50 °C for 24 h. c Disproportionation by L1 /Pd(TFA) 2 /HBpin in the absence of the regulator R . d Role of the cycloalkane in allylic dehydrogenation. Full size image Indeed, silane/borane was not found to be an essential component for isomerization or DH when an (NHC)Pd(alkyl)X equivalent was used instead of NHC/PdX 2 (e.g., [( L1 )Pd(Me)Cl] 2 , Fig. 7b ). When ( L1 )Pd(Bn)Cl was used in the absence of silane/borane and R , toluene was obtained as a byproduct instead of a conceivable BnCl via reductive elimination to Pd(0), as in other typical Pd(II)→(0)→(II) pathways. The desired product was obtained along with isomerization and disproportionation, similar to our result obtained under standard conditions in the absence of R . When all other conditions remained constant, trace amounts of products 2’ (<8%) and 3’ (<6%) were obtained from 1′a and 1′o , and 81% of the isomerization product of 1’a was observed. 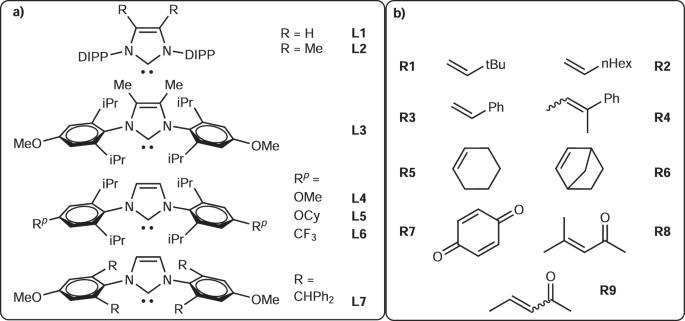Fig. 2: N-Heterocyclic carbene L and regulator R employed in this study. aNHCL1-7structures. bRegulatorR1-9structures. Again, the low 2’ productivity could be the result of missing an appropriate regulator in the system. These results suggest that an exo-to-endo isomerization step occurs before TDHA. Additionally, similar (NHC)Pd(alkyl)X performance was observed for both sets of substrates (alkyl = Bn/Me). These findings showed that (NHC)Pd(alkyl)X was an active species for endocyclic allyl CH activation (R 1 = COOMe or nPr), as was the case for methylene cyclohexane derivatives (see the Supplementary Information for details). 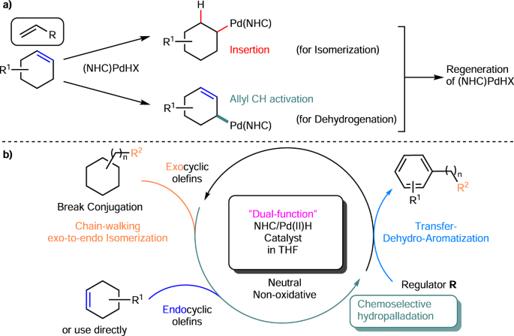Fig. 3: Catalytic action of (NHC)Pd(II)H. aCooperative steric effects of NHC and the alkene enable interchangeability of the Pd(II)H reactivity.bConversion of a mechanism consisting of undesired disproportionation and hydropalladation into the desired TDHA mechanism. Next, a comparison of the results obtained using this catalyst precursor with those obtained for our standard conditions showed that silane/borane served as a reagent only for generating (NHC)Pd(II)H from NHC/PdX 2 and not for generating (NHC)Pd(IV)H by oxidative addition. This result again showed that the role of R was to increase DH competitiveness with the undesired hydropalladations and generate a (NHC)Pd(alkyl)X species. R did not function as an acceptor for gaseous H 2 [30] ( R could not undergo reduction by gaseous H 2 in the presence of NHC-Pd(TFA) 2 without silane/borane) or to facilitate indirect (NHC)Pd(alkyl)X reductive elimination to produce Pd(0) or generate a nonhydride catalyst [9] , [10] . Thus, the 2’ : 3’ ratio decreased when the system was depleted of R or the hydropalladated 1′ and R were sterically similar (e.g., 1′e shown in Fig. 7c ). Therefore, a higher selectivity and yield were obtained by slightly increasing the quantity of R (e.g., 1′e in Fig. 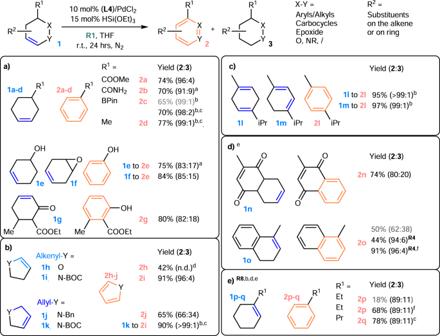Fig. 4: Endocyclic olefin 1 transfer-dehydroaromatization. aCyclohexenes.bHeterosubstituted rings.cDienes.dFused rings.eTrisubstituted alkenes. Standard conditions: The olefin (0.25 mmol),L4/PdCl2catalyst (0.025 mmol), HSi(OEt)3(0.0375 mmol), andR1(0.5 mmol) were stirred in 2 mL of THF for 24 hrs at r.t. except if otherwise indicated. The yields of2and2:3(shown in parentheses) were determined by1H NMR (average of two runs).a48 h;bas determined by GCMS (see the Supplementary Information for details);cthe standard condition shown in Fig.5was used;dpoor material balance due to a low b.p.;econversion,1o: 83; 47; 100%;1p-q: 25; 75; 89%;f50 °C. 5a ). As L n Pd(II)H can be obtained from a common (c-hexenyl)Pd(X)L n species to realize isomerization in all the relevant systems, our result suggested that the use of NHC in the absence of a strong oxidant is key to favouring the desired isomerization steps. First, the strong σ-donating ability of NHC prevented other competing steps in many other redox-active catalytic cycles, such as metallic Pd formation and Pd(II)HX reductive elimination. Pd-H oxidation was expected to be slower in the absence of a strong oxidant, and the steric hindrance of NHC increased the efficacy of chemoselective hydropalladation when employing different substrates and R (Table 1 and Figs. 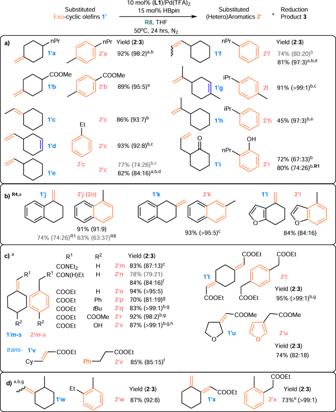Fig. 5: Exocyclic olefin 1′ transfer-dehydroaromatization. aAliphatic exocyclic olefins.bFused aromatic rings.cExo-conjugated systems.dUnsymmetric cycloisomerization products. Standard conditions: The olefin (0.25 mmol),L1/Pd(TFA)2catalyst (0.025 mmol), HBpin (0.0375 mmol), andR8(0.5 mmol) were stirred in 2 mL of THF for 24 h at 50 °C, unless otherwise indicated. The yields of2and2:3(shown in parentheses) were determined by1H NMR (as the average of two runs).a48 h;bas determined by GCMS (see the Supplementary Information for details);c60 °C;d2.5 equiv. ofR1;eOther products are from olefin isomerization;f3 equiv. ofR8;g70 °C;hwith a 9% aromatic product without OH. 4 , 5 ). Thus, hydropalladation chemistry and the quantitative analysis of the NHC effect that has been reported in the literature can serve as design guidelines. In addition, the cyclic backbone of the substrate may facilitate the desired DH. Under our standard conditions at 50 °C, acyclic olefins, such as 2-methyl-dodec-2-ene and homoallylbenzene, did not undergo DH to produce a diene as in other Pd(TFA) 2 systems (Fig. 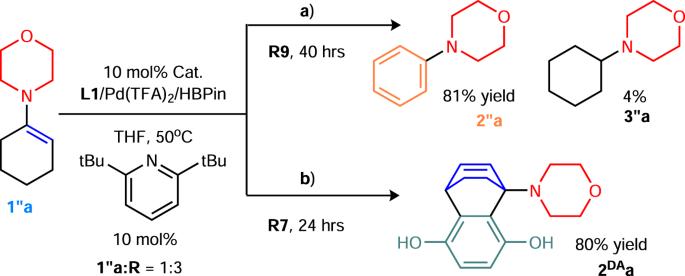Fig. 6: Catalytic synthesis of a substituted aniline and dehydrogenative Diels-Alder product. aSynthesis of a substituted aniline.bTrapping the diene for the Diels-Alder reaction. 7di–ii ). Therefore, isomerization likely occurred first in the examples using exocyclic olefins, such as allylcyclohexane (Fig. 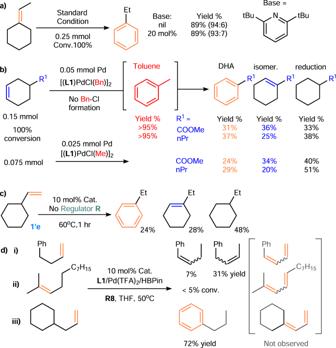Fig. 7: Control experiments and mechanistic studies. aExocyclic olefin DHA using excess base.bUsing [(L1)PdCl(R)]2as an initiator in a mimic of the CH activation step at 50 °C for 24 h.cDisproportionation byL1/Pd(TFA)2/HBpin in the absence of the regulatorR.dRole of the cycloalkane in allylic dehydrogenation. 7diii). 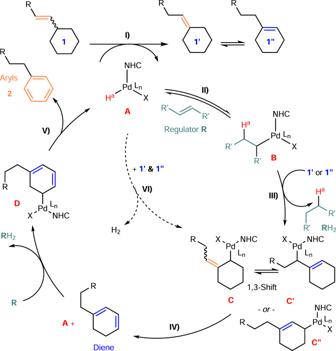Fig. 8: Proposed catalytic cycle at this stage. IChain-walking isomerization.IIChemoselective and regioselective hydropalladation of regulatorRvs.1,1′&1″.IIIH-transfer (major).IVCatalyst regeneration by isomerization and β-H elimination.VCatalyst regeneration by isomerization and β-H elimination.VIH-transfer (minor). 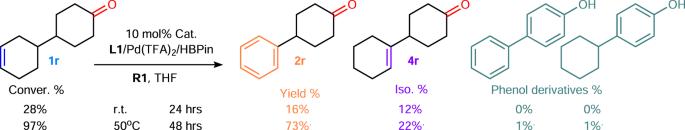Fig. 9: Chemoselective dehydrogenation. Cyclohexene vs. cyclohexanone. Figure 8 shows possible scenarios for chain-walking TDHA based on the experimental results obtained in this study and previous reports. The successful result obtained in this study was mainly attributed to the high allyl CH activation reactivity by (NHC)Pd(alkyl)X and the controlled release of (NHC)Pd(II)H (A) by the reversible hydropalladation of R . Then, the DHA step and R reduction drove the reaction forward. First, the exocyclic alkenes readily underwent exo-to-endo isomerization/chain walking ( 1 → 1′ and 1″ ) in the presence of a catalyst (A) generated from NHC/PdX 2 /silane or borane. As isomerization continued, chemoselective hydropalladation of regulator R occurred over the substrate to form species B. Next, similar to other Pd(II)/Pt(II)Me species with diimines [22] , [65] , this Pd(alkyl) species (B) ( instead of Pd(TFA) 2 ) served as an olefin ( 1′ and 1″ ) allyl CH acceptor [66] and provided the (c-hexenyl)Pd species (C/C′/C″). Therefore, a hydropalladated R reduction (H-C formation) occurred instead of the more frequent H-X formation at the end by Pd(TFA) 2 . Finally, a subsequent β -H elimination generated the diene for another CH activation, yields final product 2 , and regenerated the catalyst (A). Thus, the quantity and choice of R significantly impacted isomerization, reduction, and the transfer-DH product ratio. That is, although the additives and conditions reported in the literature (heating, as well as the use of an oxidant, alkene, and acid) were used to remove Pd-H quickly for PdX 2 catalyst regeneration [67] , the function of the R used in this study was to preserve Pd-H and regulate the desired isomerization and transfer-DH reactivity at the right time assisted by NHC. However, a pathway that utilizes A and 1′ / 1″ to form molecular H 2 may still be possible at high temperature. Fig. 8: Proposed catalytic cycle at this stage. I Chain-walking isomerization. II Chemoselective and regioselective hydropalladation of regulator R vs. 1 , 1′ & 1″ . III H-transfer (major). IV Catalyst regeneration by isomerization and β-H elimination. V Catalyst regeneration by isomerization and β-H elimination. VI H-transfer (minor). Full size image A comparison of the proposed DH catalytic cycles of olefins by (NHC)Pd(II)H and cyclohexanone by PdX 2 [13] , [14] , [15] , [20] showed that a highly chemoselective DH of cyclohexene over cyclohexanone is possible (Fig. 9 ). This reaction occurred because NHC can suppress Pd(II)HX reductive elimination and block the DH pathway based on PdX 2 and Pd(enolate)X. As a result, 1r underwent chemoselective DH to produce 2r and yield <2% phenol/cyclohexenone (~73:2 or 97:3). This chemoselectivity was useful because existing DH methods based on using PdX 2 at a higher temperature or under acidic conditions mostly favor cyclohexanones or both phenol and cyclohexenone. Thus, the 1′i DH to produce a phenol shown in Fig. 5a was likely initiated by allyl isomerization, not by ketone DH catalyzed by soluble Pd nanoparticles [23] . Fig. 9: Chemoselective dehydrogenation. Cyclohexene vs. cyclohexanone. Full size image In summary, the unwanted Pd-H species produced in most previous dehydrogenative aromatization catalytic cycles were repurposed as an active catalyst by NHC to carry out both olefin chain-walking isomerization and transfer-(de)hydrogenation. Both endocyclic olefins and many easily accessible exocyclic olefins were found to act as effective DHA substrates in the presence of logical combinations of (NHC)Pd(II)HX and a regulator R . This change in the active DH species resulted in good reactivity and functional group tolerance under redox-neutral and mild conditions and provided a basis for the chemoselective DH of an allyl CH instead of other highly competitive CHs next to ketone and N-sites by removing the PdX 2 species in the catalytic cycle. Using Pd-H species also obviated the oxidative and high-temperature conditions regularly employed in related redox-active catalytic cycles using common oxidants, which should be useful for late-stage aromatization. The dual-function catalyst also enabled us to make a synthetic advance that bypassed the challenges associated with incomplete exo-to-endo isomerization and tedious separation of structurally similar olefins using stepwise approaches. Overall, this study demonstrates the potential of exploiting NHC effects to regulate the reactivity of highly competitive hydrometallation and allyl CH activation. Explorations of transfer-hydrogenation using cyclohexenes as nonpolar H-donors and other transformations that involve exo-to-endo isomerization are now underway. General procedure for TDHA 1 or 1′ (0.25 mmol) and R (0.50 mmol) were added to an NHC/PdX 2 catalyst mixture (0.025 mmol) with a hydride source (0.0375 mmol) in 2 mL of THF, and the resulting mixture was stirred for the indicated time period at the indicated temperature. The yield and selectivity were then determined by 1 H NMR or GCMS (as the average of two runs). The product structures were confirmed by isolation.